A novel metatranscriptomic approach to identify gene expression dynamics during extracellular electron transfer Microbial respiration via extracellular electron transfer (EET) is a ubiquitous reaction that occurs throughout anoxic environments and is a driving force behind global biogeochemical cycling of metals. Here we identify specific EET-active microbes and genes in a diverse biofilm using an innovative approach to analyse the dynamic community-wide response to changing EET rates. We find that the most significant gene expression responses to applied EET stimuli occur in only two microbial groups, Desulfobulbaceae and Desulfuromonadales . Metagenomic analyses reveal high coverage draft genomes of these abundant and active microbes. Our metatranscriptomic results show known and unknown genes that are highly responsive to EET stimuli and associated with our identified draft genomes. This new approach yields a comprehensive image of functional microbes and genes related to EET activity in a diverse community, representing the next step towards unravelling complex microbial roles within a community and how microbes adapt to specific environmental stimuli. Extracellular electron transfer (EET) is a process whereby microbes are able to respire by moving electrons outside of the cell to reduce solid-phase electron acceptors [1] , [2] . The ability of microbes to electronically interact with solid-phase electron acceptors is a widespread phenomenon that drives geochemical cycles around the globe and has changed the way we view microbial respiration [3] , [4] , [5] . The first EET-capable microbes described were Shewanella and Geobacter [1] , [2] , and the study of these pure cultures has led to the description of three different EET mechanisms: outer membrane-bound multi-haem c -type cytochromes [1] , [2] , [6] ; soluble electron carriers [7] ; and conductive bacterial nanowires and/or extracellular matrices [8] , [9] . In nature, it is likely that EET occurs as a result of community processes arising from complex multi-species metabolic interactions [10] . In such diverse communities it is difficult to understand which taxa (and which genes) are involved with EET, and how the community responds to environmental changes that impact EET [11] . Therefore, the objective of our study was to address specific EET-active microbes and genes within a diverse community and evaluate responses to changing EET conditions. To accomplish this objective, we applied a dynamic metatranscriptomic approach to assess community response to specific stimuli expected to alter the EET activity of a complex microbial community. For any microbial community it is important to understand the genetic potential, functional activity and functional adaptability in response to environmental changes. To this point, metagenomic analyses have been used to define both taxonomic and the collective gene pool contents of many natural communities [12] , [13] , while metatranscriptomic approaches have provided gene expression profiles from microbial communities in many different environments [14] , [15] , [16] , [17] . However, in natural systems it is difficult to ascribe function to specific microbial groups, as the genetic background can shift temporally (for example, day versus night [17] ) and/or spatially (for example, depth profiles [14] ). Furthermore, while environmental data are regularly collected during these studies, the interpretation of community data is often challenged by multiple variables changing simultaneously, making it difficult to extract specific microbes and genes that are responding to a given variable or stimulus. To achieve our objectives relative to EET-related communities, we developed a method to analyse the dynamics of community-wide transcription in response to a specific EET stimulus within a biofilm community of the same genetic background. We conducted a sequential metatranscriptomic analysis of a functionally stable, taxonomically diverse, EET-active microbial community [18] exposed to increasing and decreasing EET rates in a microbial fuel cell (MFC). MFCs have been demonstrated as useful tools to evaluate EET reactions at electrode surfaces, which can act as analogues to environmental solid-phase electron acceptors [11] . Using a combination of bioelectrochemical, metagenomic and metatranscriptomic approaches, we acquired a comprehensive data set enabling us to link physiological function to specific microbes and genes within the EET-active community. Bioelectrochemical response to changing EET rates We operated a MFC regularly fed with wastewater for 2 years [18] . Wastewater was chosen as a feed-stock because it contains diverse microbial populations and variable substrates that can be used for microbial fermentation, anaerobic respiration with soluble electron acceptors and EET respiration with the solid electrode. Using this MFC community, we subjected the electrode-associated biofilm to three sequential operational changes ( Fig. 1 ): baseline condition related to static EET activity (MFC); increased EET rates achieved by set-potential (SP) conditions that made the electrode surface a more electropositive (better) electron acceptor; and decreased EET rates achieved by open-circuit (OC) operation, which stopped electron flow through the circuit and limited EET activity at the electrode. Electrochemical measurements were collected during each condition. The MFC operational condition (S0) showed an anodic current density of 70 mA m −2 at an operating anodic potential of approximately −280 mV versus standard hydrogen electrode (SHE), and an electron recovery efficiency of ~20%. These performance metrics were reproducibly observed throughout the 2-year operation of the MFC system [18] . The potentiostatic operation (S1), with the anodic potential controlled to +100 mV versus SHE allowed for the measurement of anodic microbial activity independent of system limitations [18] , [19] , resulted in a current density that was 8 times higher (550 mA m −2 ) than that observed for the MFC condition, and the electron recovery efficiency was ~50%. During the OC condition (S2) the anode electrode was disconnected from the cathode electrode and operated with zero current production and 0% electron recovery. The evaluation of genomic and transcriptomic responses to each of the stimuli (S1 and S2) was conducted from biofilm samples collected after each operational change had stabilized for 45 min. 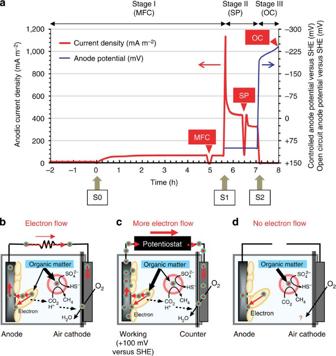Figure 1: Operational data and schematic of sampling conditions. (a) Current and/or voltage responses throughout the different sampling conditions. Reactor anolyte replacement (wastewater replacement) occurred at S0 under MFC conditions. The condition was changed from MFC operation (b) to SP operation (c) at S1. The anode potential was controlled to +100 mV versus SHE using a potentiostat during SP operation. The operational condition was changed from SP to OC at S2. During the OC condition there was no connexion between the anode and cathode resulting in zero current (d). DNA and RNA extraction were conducted using samples collected during all three operating conditions: MFC after 5 h from S0, SP after 45 min from S1 and OC after 45 min from S2. Figure 1: Operational data and schematic of sampling conditions. ( a ) Current and/or voltage responses throughout the different sampling conditions. Reactor anolyte replacement (wastewater replacement) occurred at S0 under MFC conditions. The condition was changed from MFC operation ( b ) to SP operation ( c ) at S1. The anode potential was controlled to +100 mV versus SHE using a potentiostat during SP operation. The operational condition was changed from SP to OC at S2. During the OC condition there was no connexion between the anode and cathode resulting in zero current ( d ). DNA and RNA extraction were conducted using samples collected during all three operating conditions: MFC after 5 h from S0, SP after 45 min from S1 and OC after 45 min from S2. Full size image Metagenomic analyses Both DNA and RNA were coextracted from the three different samples of the anode-associated biofilm. DNA and RNA were then separated and sequenced for each sample described above (MFC, SP and OC). We analysed both DNA and mRNA sequences, followed by in silico analyses of our metagenomic assembly and read mapping of DNA and mRNA to the assembled contigs ( Fig. 2 ). 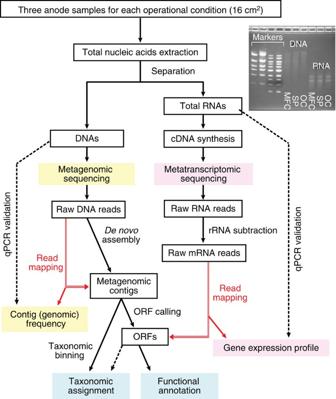Figure 2: Schematic of the experimental and analytical workflow. DNAs and total RNAs of three conditions after separation are shown. Figure 2: Schematic of the experimental and analytical workflow. DNAs and total RNAs of three conditions after separation are shown. Full size image Our metagenomic assembly ( Supplementary Table S1 ) yielded 224,995 contigs. The JCVI prokaryotic metagenomic (MG) pipeline [20] was used to call open reading frames (ORFs) and resulted in 445,806 ORFs identified, and 304,439 ORFs (68.2%) were assigned to KEGG IDs with functional and taxonomic information. The KEGG Automated Annotation Server (KAAS) [21] was used to assign 179,677 ORFs (40.3%) to a KEGG Orthology (KO) [22] for metabolism analyses. All 445,806 genes (ORFs) associated with the assembled contigs were evaluated separately to determine their taxonomic classification using the JCVI MG pipeline [20] . During this process, taxonomic misassignments can frequently occur because of horizontal gene transfer, lack of reference sequence for the specific taxonomic group, or highly variable genes; however, a single taxon should be associated with one contig. The results of our taxonomic binning method for contig classification led to 375,698 ORFs (84%) assigned to Kingdom, 354,591 ORFs (80%) assigned to Phylum, 330,090 ORFs (74%) assigned to Class , 319,827 ORFs (72%) assigned to Order, and 306,930 ORFs (69%) assigned to Family, respectively. Our contig taxonomic assignment method increased the taxonomic assignments to ORFs relative to the JCVI MG pipeline and provided the opportunity to use the contig taxonomic assignments to determine bin-genome associations. Over 60% of raw DNA sequence reads mapped to our metagenomic contigs ( Supplementary Table S2 ). This read-mapping metric was used to obtain relative DNA frequencies within the community as determined by DNA-RPKM values, where RPKM indicates reads per kilobase per million mapped reads [23] . From the 16,569,236 raw DNA reads that mapped to metagenomic ORFs, 15,875,153 reads (95.8%) were mapped to only one specific ORF. The non-specifically mapped reads were most likely associated with highly conserved regions in a wide variety of microbial genomes, repeat regions within a single microbial genome, or a misassembly that created duplicated regions in the contigs/ORFs. The fluctuation of contig frequency among the three operational conditions (MFC, SP and OC) was evaluated using scatter plots of DNA-RPKMs associated with each contig between two operational conditions ( Supplementary Fig. S1 ). The correlation coefficients were calculated as 0.976 between conditions MFC and SP, and 0.961 between conditions SP and OC. The plots indicate that a small taxonomic fluctuation is observed across the three operational conditions, which were originally sampled from different locations of the anode biofilm. However, the taxonomic heterogeneity between these samples was very small, indicating a similar genetic background for the three spatially separated biofilm subsamples. This enabled the use of an average DNA-RPKM value for determining mRNA/DNA ratios for gene expression profiles of the static community and across multiple condition changes. Bin-genome analyses To analyse the taxonomic composition of the EET-related microbial community, we conducted both metagenomic analyses (based on DNA-RPKM values) and 16S rRNA clone analyses (based on clones associated to a taxon per total clones sequenced) of both the Bacterial and Archaeal communities ( Supplementary Fig. S2 ). These different analytical strategies showed a reasonable correlation between the two types of genomic analyses. The results clearly indicate that Deltaproteobacteria and Euryarchaeota were the dominant groups within the community. A higher resolution analysis revealed three dominant Deltaproteobacteria subcategories, including family Desulfobulbaceae , family Desulfobacteraceae and order Desulfuromonadales . The Euryarchaeota in the EET-active community was occupied solely by family Methanosarcinaceae . A strain-level analysis was executed by identifying the assembled metagenomic contigs related to dominant strains within these four taxonomic groups. DNA frequency plots of the contigs (contig length versus DNA-RPKM) for the four dominant taxa showed clearly defined clusters associated with the longer contigs, which are associated with potentially abundant strains ( Supplementary Fig. S3 ). A more comprehensive clustering analysis was performed on the contigs by using these DNA frequency levels (DNA-RPKM), taxonomic assignments, contig length (bp) and GC content (%) ( Fig. 3 ). This clustering analysis enabled draft genome association to four different highly abundant strains (bin-genomes) that may be directly related to EET activity. The bin-genomes were identified as strains DB1 and DB2 in family Desulfobulbaceae , DF1 in family Desulfobacteraceae and MS1 in family Methanosarcinaceae ( Fig. 3 ). The basic information of the four bin-genomes is summarized in Table 1 , and the clustering criteria are listed in Supplementary Table S3 . 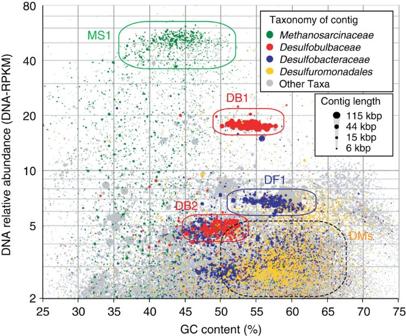Figure 3: Bin-genomes of dominant strains within the EET-active microbial community. Bin-genome clusters (MS1, DB1, DB2 and DF1) were established using the estimated taxonomic classification of contigs (colour of dots), contig lengths (size of dots), GC content of contigs (%) and contig relative frequency (DNA-RPKM). Figure 3 also shows a loose clustering of contigs assigned to order Desulfuromonadales . Even though the contigs related to Desulfuromonadales did not reveal a strain -level bin-genome, we assigned these contigs to group DMs and included this group in our subsequent gene expression analyses because the order includes the model genus Geobacter [1] , [2] . Figure 3: Bin-genomes of dominant strains within the EET-active microbial community. Bin-genome clusters (MS1, DB1, DB2 and DF1) were established using the estimated taxonomic classification of contigs (colour of dots), contig lengths (size of dots), GC content of contigs (%) and contig relative frequency (DNA-RPKM). Full size image Table 1 Summary of bin-genomes associated by contigs clustering. Full size table To validate that the four hypothesized bin-genomes were associated with unique strains, we compared their phylogenetic positions and abundance frequencies to those from the 16S rRNA clone library analysis. Full length 16S rDNA genes were not observed in the bin-genomes because it is difficult to assemble contigs for such highly conserved regions. Therefore, we used other single copy marker genes such as dsrA [24] (also a marker for dissimilatory sulphate reducers) and gyrB [25] , [26] for Deltaproteobacteria , and mcrA [27] (also a marker for methanogens) for Methanosarcinaceae . A comparison of the dsrA-, gyrB- and mcrA- based phylogenetic trees revealed significant correlations, for both phylogeny and abundance, between the relatively abundant phylotypes in the 16S rRNA analysis and the dominant bin-genomes in the metagenomic analysis ( Supplementary Figs S4–S6 ). Genomic parameters of the four bin-genomes were also compared with closely related complete chromosomes. Bin-genomes DB1 and DF1 showed over 90% completeness based on single copy gene catalogues, while bin-genomes DB2 (88% completeness) and MS1 (85% completeness) showed lower draft genome quality because of the poor assembly for MS1 and low RPKM value for DB2 ( Supplementary Tables S4–S6 ). These comparative analyses indicated that our bin-genomes represent unique and dominant strains within their respective families, which lends further confidence to our metagenomic data set used for subsequent dynamic metatranscriptomic analyses. Metatranscriptomic analyses Approximately 95% of the raw RNA reads were discarded based on results from a tera-blastn search against the SILVA database [28] . The remaining 5% of the raw RNA reads were retained as mRNA reads for subsequent read mapping analyses. The raw mRNA reads from each operational condition were mapped to the metagenomic contigs/ORFs to analyse gene expression profiles ( Supplementary Table S2 ). These analyses showed that ~60% of the raw mRNA reads mapped to the contigs, similar to the read mapping results using raw DNA reads. The relative abundance of mRNA within the community was determined by mRNA-RPKM [23] . A total mRNA-RPKM of 1,471,844 was observed for condition MFC, 1,488,979 for condition SP and 1,489,275 for condition OC. We found that 124,466 ORFs, out of 445,806 total ORFs (28%), were transcribed during at least one condition and were treated as coding sequences (CDSs). The full data set containing all gene expression profiles relative to all ORFs is too large (79 MB) to be shown; therefore, we will provide the data set via personal request. Microbial taxa responding to EET stimuli The taxonomic groups responding to changing EET rates were evaluated by enumerating community gene content (DNA-RPKM) and gene expression (mRNA-RPKM), and comparing these values across the different conditions. These data revealed that only two taxonomic groups, Deltaproteobacteria and Euryarchaeota , had high gene expression levels relative to the DNA frequency, which suggests that those two taxa were relatively active in the community ( Fig. 4a ). Within those taxa, strains DF1 and MS1 were the most active over all conditions; however, gene expression dynamics indicated that strains DF1 and MS1 were not specifically responsive to EET-related changes ( Fig. 4b ). On the other hand, the most significant gene expression changes occurring as a result of the different operational conditions (SP and OC) were associated with the group DMs and strain DB1, both contained within class Deltaproteobacteria ( Fig. 4b ). This result suggests that these taxa were directly involved with EET-related activity. 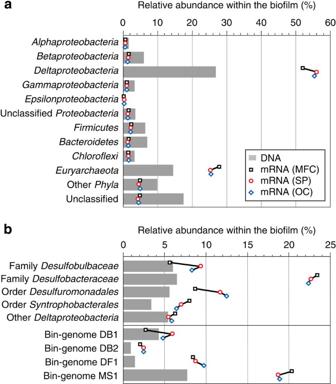Figure 4: Relative abundance of DNA and mRNA within the EET-active biofilm. (a) Phylum-level classification except forProteobacteria, which is divided to class level. (b)Deltaproteobacteriadivided to family-or order-level classification, and the four strains. Metatranscriptomic and metagenomic data were analyzed for samples collected from three operational conditions (MFC, SP and OC). Figure 4: Relative abundance of DNA and mRNA within the EET-active biofilm. ( a ) Phylum-level classification except for Proteobacteria , which is divided to class level. ( b ) Deltaproteobacteria divided to family-or order-level classification, and the four strains. Metatranscriptomic and metagenomic data were analyzed for samples collected from three operational conditions (MFC, SP and OC). Full size image Highly responsive genes related to EET stimuli The gene expression fold change for each CDS was evaluated as a function of operational condition change using scatter plots of mRNA-RPKMs ( Fig. 5a ). The scatter plots clearly show that gene expression for CDSs assigned to strain DB1 and group DMs was significantly changed in response to the EET stimuli, whereas strains DF1 and MS1 did not show significant gene expression differences between the two operational conditions. 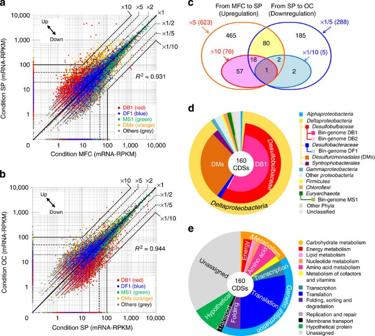Figure 5: Genes responding to operational changes. Scatter plots of all CDS responses as measured by mRNA frequency (mRNA-RPKM) between MFC and SP conditions (a), and between SP and OC conditions (b). Strains DB1, DF1, MS1 and group DMs are shown as unique colours, all other groups are shown in grey. (c) Detailed summary of CDSs that showed a significant response to changing EET rates. The 160 significantly changed CDSs were analyzed relative to taxonomic assignment (d) and KO-based functional annotation (e). Figure 5: Genes responding to operational changes. Scatter plots of all CDS responses as measured by mRNA frequency (mRNA-RPKM) between MFC and SP conditions ( a ), and between SP and OC conditions ( b ). Strains DB1, DF1, MS1 and group DMs are shown as unique colours, all other groups are shown in grey. ( c ) Detailed summary of CDSs that showed a significant response to changing EET rates. The 160 significantly changed CDSs were analyzed relative to taxonomic assignment ( d ) and KO-based functional annotation ( e ). Full size image To address the important genes related to EET activity in the community, we closely evaluated those CDSs that showed a significant expression change (≥5-fold and ≥10-fold change) between operational conditions listed in Supplementary Data 1 . The CDSs that had mRNA-RPKM values lower than 20 for both conditions were treated as low-quality CDSs, and not used for this analysis to extract CDSs that showed a significant expression change. We identified the upregulated CDSs from condition MFC using two criteria for ‘highly’ upregulated genes with ≥10-fold upregulation (or from zero to over 100), and for ‘moderately’ upregulated genes with ≥5-fold upregulation (or from zero to over 50) ( Fig. 5a ). We also identified the downregulated CDSs from condition SP to condition OC using two criteria for significant fold changes that included downregulation of over 100 to zero, or over 50 to zero, respectively ( Fig. 5b ). Out of 810 total CDSs showing a 5- or 10-fold change in expression levels, we found that 160 CDSs (≥10-fold change under at least one condition change or ≥5-fold changes under both condition changes) appeared to have a significant expression change when exposed to the SP or OC conditions ( Fig. 5c ), suggesting that these CDSs were involved with EET processes from the microbes to the electrode. For these 160 CDSs, the taxonomic classification was analysed based on contig level taxonomic assignment ( Fig. 5d ), while the functional annotation was analysed based on KEGG BRITE hierarchy ( Fig. 5e ). Figure 5d shows that a majority of the significantly changed CDSs were assigned to strain DB1 and group DMs, which implies that these taxa were specifically related to EET activity in the community. Figure 5e shows that the KO-based functional annotations of these CDSs were related to genetic information or unassigned functions. Notably, we found two gene clusters (contig_301860, position 2453–5506 and contig_63633, position 20700–23863) belonging to strain DB1 that changed by 100-fold upregulation when exposed to the SP condition while the average gene expression change in strain DB1 was only 1.6-fold upregulation for this condition change. These two gene clusters are likely important for the strain to adapt to a higher EET rate. However, it was not possible to functionally annotate most of the associated CDSs. Gene expression dynamics related to anaerobic respiration Specific metabolic pathways were analysed relative to the whole community and the dominant bin-genomes under the baseline condition (MFC), as well as changing EET conditions (SP and OC). The selected pathways included key gene families related to energy metabolism, cell activity, c -type cytochromes and competitive anaerobic respiration pathways including sulphate reduction, nitrate reduction and methanogenesis. 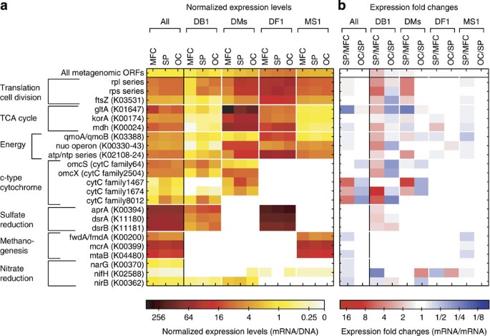Figure 6: Overall gene expression levels and dynamics related to anaerobic respiration. (a) The static overview of the whole community gene expression levels for each condition and abundant microbial groups. (b) Gene expression changes between two operational conditions for selected anaerobic respiration-related gene families. Figure 6a shows the gene expression levels normalized to DNA abundance (mRNA/DNA) for all three operational conditions. This view offers a snapshot of the community function relative to each condition and indicated high activities associated with sulphate reduction, mainly conducted by Desulfobacteraceae strain DF1 [24] , and methanogenesis, mainly conducted by Methanosarcinaceae strain MS1 [27] . However, little activity appeared to be associated with EET-related pathways for these strains, as shown by the lower gene expression levels for c -type cytochromes compared with those potentially competitive respiration pathways within the community. Figure 6: Overall gene expression levels and dynamics related to anaerobic respiration. ( a ) The static overview of the whole community gene expression levels for each condition and abundant microbial groups. ( b ) Gene expression changes between two operational conditions for selected anaerobic respiration-related gene families. Full size image Interestingly, when the fold change of these same gene families were analysed (mRNA/mRNA), it was clearly evident that c -type cytochrome gene families experienced the highest levels of expression change relative to the other respiration pathways ( Fig. 6b ). This dynamic view of gene expression offers insight into the immediate adaptive response within the community as it relates to EET. Only strain DB1 and group DMs were immediately responsive to EET stimuli, and the significantly changed genes were those related to c -type cytochromes. Other gene families that showed significant responses for both strain DB1 and group DMs included ftsZ for cell division, ribosomal proteins for translation and NADH dehydrogenases for electron transport to the inner membrane quinone pool (only for strain DB1), which suggests that these microbes activated genes for adapting to new environmental conditions. The c -type cytochrome trends also suggest that group DMs and strain DB1 used different c -type cytochromes to facilitate high EET rates. The outer membrane multi-haem c -type cytochromes OmcS and OmcX have been reported as important proteins for EET reactions in Geobacter strains [1] , [29] , [30] ; however, the other c- type cytochrome families showing the highest expression changes in our study have not been functionally characterized. Notably, gene expression related to sulphate reduction in the strain DF1 and methanogenesis in the strain MS1 was completely unchanged in response to EET stimuli. A detailed description of these results can be found in Supplementary Table S7 and Supplementary Fig. S7 . Quantitative validation of metagenomic and metatranscriptomic analysis A quantitative validation of metagenomic and metatranscriptomic analyses is necessary to achieve a higher confidence in the data. To validate our metagenomic and metatranscriptomic analyses, quantitative PCR (qPCR) was performed for six key metabolic genes found to be associated with the dominant bin-genomes DB1, DF1 and MS1, and one significantly changed hypothetical gene from DB1 ( Supplementary Table S8 ). This analysis demonstrated consistency between our qPCR (copies per ng DNA or pg RNA) and metagenomic/metatranscriptomic results (RPKM) ( Fig. 7 ). Correlation coefficients of R 2 =0.94 and R 2 =0.88 were found for metagenomic and metatranscriptomic data, respectively. 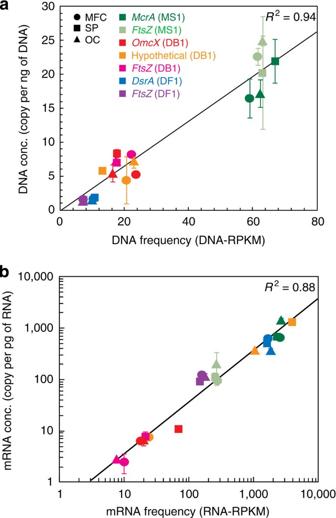Figure 7: Comparison of quantitative PCR and metagenomic and transcriptomic data. (a) The relationship between qPCR of DNA (copy number) and metagenomic DNA frequency (DNA-RPKM). (b) The relationship between qPCR of cDNA produced from RNA (copy number) and mRNA frequency (mRNA-RPKM). Circle, condition MFC; square, condition SP; triangle, condition OC. The targeted ORFs are described inaandSupplementary Table S8. The data are presented as mean±s.d. obtained from three separated trials. The approximation curve and the correlation coefficient (R2) are given. Figure 7: Comparison of quantitative PCR and metagenomic and transcriptomic data. ( a ) The relationship between qPCR of DNA (copy number) and metagenomic DNA frequency (DNA-RPKM). ( b ) The relationship between qPCR of cDNA produced from RNA (copy number) and mRNA frequency (mRNA-RPKM). Circle, condition MFC; square, condition SP; triangle, condition OC. The targeted ORFs are described in a and Supplementary Table S8 . The data are presented as mean±s.d. obtained from three separated trials. The approximation curve and the correlation coefficient ( R 2 ) are given. Full size image Metagenomic and metatranscriptomic analyses have enabled researchers to begin assessing microbial gene pools and functions even if the microbes have not been isolated or cultivated. However, assigning function to a specific taxon, and exclusively identifying functional pathway responses to environmental stimuli within a community has not yet been comprehensively reported. We applied DNA sequencing with metagenomic assembly, constructed draft genomes, annotated the taxonomy and function of the ORFs, and subsequently performed read mapping of mRNA sequences to the metagenomic ORFs. Generally, this approach improves the number of mRNA reads used for analyses because they are mapped to an identical DNA template [31] , [32] , [33] , [34] . Additionally, this procedure allowed us to correlate gene expression results to specific strains in the community. This enabled the discovery of new microbial strains and associated gene targets, which might relate to key proteins for community function ( Fig. 2 ). Here we report a systems biology study that successfully unifies bioelectrochemical ( Fig. 1 ), metagenomic ( Fig. 3 ) and metatranscriptomic ( Figs 4 , 5 , 6 ) data sets to identify the responsive strains (draft genomes) and functional EET-related genes in a diverse community. The success of this approach relies heavily on using simplified EET stimuli to induce gene expression changes, and the strength of using the same genetic background for metatranscriptomic analyses. Generally, metatranscriptomic analyses have demonstrated between 0.5 and 40% of mRNA reads mapped [15] , [16] , [31] , [32] , [33] , [34] , [35] , [36] , [37] . We found that over 60% of mRNA reads were mapped to the reference metagenomic contigs ( Supplementary Table S2 ), which indicates a higher representation of overall gene expression profiles within the microbial community. Additionally, we have quantitatively validated our metagenomic and metatranscriptomic results using qPCR ( Fig. 7 ), giving greater confidence in our findings. The detailed discussion for the method development can be found in Supplementary Discussion . Our static versus dynamic analyses of community function revealed that gene expression normalized to gene abundance may not comprehensively describe the activity of a given community in response to stimuli ( Fig. 6 ). Our EET-related microbial community harboured an abundance of sulphate reducers and methanogens that were consistently active within the community as analysed by the mRNA/DNA ratio (static view, Fig. 6a ); however, the sulphate reduction and methanogenesis pathways were not immediately responsive to EET-related stimuli as analysed by the mRNA/mRNA ratio (dynamic view, Fig. 6b ). These data indicate that an analysis of gene expression dynamics across multiple conditions for a stable metagenome can identify specific functional pathways. In a future study we will explore the temporal effects for the community-wide gene expression dynamics as they relate to EET stimuli. The dynamic view of gene expression profiles revealed the correlation of EET activity to specific pathways, and specific microbial strains DB1 and DMs, within the diverse biofilm community. The observed microbe–electrode responses were immediate reactions to the applied EET stimuli (after 45 min). However, this does not preclude the possibility that microbe–microbe responses do occur and may be observable after longer time periods. Notably, strain DB1 was identified as the most EET-active microbe and assigned to family Desulfobulbaceae ( Fig. 4b ). Recently, a strain from the family Desulfobulbaceae has been identified as an important group for EET-related activity in marine sediments, which couples spatially separate biogeochemical processes via EET reactions [38] . Interestingly, the bin-genome DB1 featured a high number of genes encoding multi-haem c -type cytochromes associated with genus Geobacter , although strain DB1 is not phylogenetically associated to the family Geobacteraceae . Some of the responsive genes to EET stimuli included homologous genes of omcX and omcS, which are known to be related to EET activity in the Geobacter strains [1] , [29] , [30] ; additionally, we observed two other highly responsive uncharacterized c -type cytochromes (families 1674 and 8012) when EET stimuli were applied ( Fig. 6b ). This finding is the first report of Geobacter -like c -type cytochromes existing and functioning as a part of enhanced EET activity within the family Desulfobulbaceae. The dynamic gene expression trend of the dissimilatory sulphate reduction pathway in strain DB1 showed that upregulated genes remained at similar expression levels from condition MFC to condition SP, relative to the whole DB1 transcriptome. Further, downregulation of these genes was not observed during the change from condition SP to condition OC ( Fig. 6 ). This trend suggests that dissimilatory sulphate reduction was not affected by electrode potential changes; however, sulphate reduction was consistently performed even when EET rates fluctuated. The average gene expression change for the bin-genome DB1 showed a 1.6-fold upregulation under the SP condition, and a 0.8-fold downregulation under the OC condition. We observed two gene clusters in the bin-genome DB1 that had upregulations over 100-fold in response to higher EET rates (SP) ( Fig. 5a ), and downregulation below 0.6-fold in response to zero current condition (OC) ( Fig. 5b ). The significant expression changes suggest that these two previously undescribed gene clusters associated with strain DB1 may be very important for community adaptation to EET changes and are therefore future targets for more in-depth EET-related studies of strain DB1. The detailed discussion for the strain DB1 and group DMs functions within the community can be found in Supplementary Discussion . In summary, we have developed a new approach with two major strengths that led to new EET insights. These strengths include the ability to simplify stimuli (specific to EET in this case), and the ability to maintain the same genetic background throughout the application of stimuli. These two concepts may be applied to a variety of laboratory or field studies to determine microbial responses to induced stimuli. Consequently, our systematic approach significantly improved in silico data analyses relative to previous reports, and enabled the identification of the central genes relating to EET via comparative gene expression profiles within a complex microbial community. Overall, these results provide a next step towards unravelling the complex microbial interactions that are required for community adaptation to environmental EET stimuli. EET stimuli for dynamic metatranscriptomic experiments A MFC used for municipal wastewater treatment was operated for over 800 days under repeat-batch mode with electricity recovery from organic matter in the wastewater [18] . The MFC configuration and long-term operating condition are described in the Supplementary Methods . A fresh primary clarifier sample collected from North City Water Reclamation Plant (San Diego, CA, USA) was added the MFC before executing the operational changes. The chemical oxygen demand of the fresh primary clarifier sample was 333 mg l −1 on 16 December 2010), which was determined using a potassium chromide assay according to the manufacturer’s instructions (Orion CODHP0, Thermo Scientific). This sample was introduced to the starved MFC community, where the chemical oxygen demand was 45.3 mg l −1 (condition MFC, Fig. 1b , stimulus S0 at 0 h). After 5 h of operation, one-third (16 cm 2 ) of the carbon cloth electrode was collected from the anodes by ethanol-sterilized scissors in an anaerobic glove box, immediately frozen by liquid nitrogen and stored in a −80 °C freezer. After a 30-min recovery period from the MFC operation sampling, the anode potential was controlled to +100 mV versus SHE using a potentiostat (HA-151A, Hokuto Denko) and an Ag/AgCl reference electrode (condition SP, Fig. 1c , stimulus S1 at 5.5 h). A sample was collected 45 min after current stabilization was observed under the SP condition and was used to analyse the gene expression profile occurring during the higher current-generating condition. The same size of anode (16 cm 2 ) was collected and stored after treatment as described above. After another 30-min recovery phase from the SP sampling, the anode electrode was disconnected from the cathode electrode and operated under OC conditions with zero current production and 0% electron recovery (condition OC, Fig. 1d , stimulus S2 at 7.25 h). The OC anode potential versus SHE (mV) was determined relative to an Ag/AgCl electrode. The last anode sample, reflecting the gene expression profile during the zero current condition, was collected 45 min after the operational change was made when the anode potential was observed to be stable around −230 mV versus SHE (condition OC). A similar size of anode (16 cm 2 ) was collected and stored as described above. Sequencing and assembly Both DNA and RNA of the anode-associated microbiome were coextracted using a MObio PowerBiofilm RNA Isolation Kit with some modification of the manufacturer’s instructions to achieve the highest yield of total nucleotide. Extracted total nucleotide was separated using the AllPrep DNA/RNA Mini Kit (Qiagen). The prepared DNA was used for library construction for Illumina and 454 sequencing, 16S rRNA clone library analysis and qPCR. Total RNA was treated with Turbo DNA free (Ambion) to completely remove contaminating DNA, randomly fragmented to ~200–300 nt in length, then used for cDNA library synthesis for cluster generation and sequencing. Paired-end and fragment libraries for DNA and cDNA were prepared following Illumina’s protocol, with a few exceptions. Cluster generation and sequencing were conducted using the Genome Analyzer IIx (Illumina, GAIIx), employing the 101-bp read length option. Both fragment and paired-end sequencing approaches were conducted by Illumina’s standard protocol [39] . Mated-pair library construction (3-kb insertion size), emPCR, enrichment and 454 sequencing on the 454 Titanium FLX (Ti-FLX) platform were performed following the vendor’s standard operating procedures with some modifications [39] . Mated-pair 454 DNA sequencing was conducted in addition to paired-end Illumina to yield longer reads that could be assembled into longer contigs. The de novo assembly of metagenomic sequences was conducted using a multi-step process ( Supplementary Table S1 ). The detailed methods for sequencing and assembly steps are described in the Supplementary Methods . The assembled contigs from this metagenomic study have been deposited at DDBJ/EMBL/GenBank under the accession AMWB00000000 . The version described in this paper is the first version, AMWB01000000 . ORF calling and functional annotation Contigs produced by de novo assembly were processed with the JCVI prokaryotic metagenomic ORF calling & annotation pipeline described elsewhere [20] (details in Supplementary Methods ). For the KO group assignment [22] , we used the KAAS [21] with the BBH (bi-directional best hit) method set to 45 as the threshold assignment score. Clusters of orthologous groups [40] were converted from the KO assignment. Proteins were considered as c- type cytochromes if their sequence contained at least one CXXCH motif for covalent haem [41] . Each predicted c- type cytochrome ORF was assigned the c- type cytochrome family ID constructed by Butler et al. [29] of the best BLAST hit retrieved from the Geobacter c- type cytochromes using an e-value cut-off of 1e −6 (details in Supplementary Methods ) [42] . Taxonomic classification of contigs According to our method for contig classification of the taxonomic assignment, if more than 50% of the genes within a contig were attributed to the same Kingdom, the contig and all related genes in the contig would be assigned to that Kingdom. Phylum and Class level NCBI (National Center for Biotechnology Information) taxonomies were assigned using the same threshold of more than half of the genes matching to the same taxon. For Order- and Family-level classifications, the criteria were changed so that more than 40% for the Order-level and 34% for the Family-level taxonomy. Subtraction of rRNA from total RNA The raw Illumina RNA sequence data files were converted from fastq to fasta format and then aligned against the SILVA (SSURef and LSURef) database, build 106 (April 2011) ( [28] ), using tera-blastn on Decypher Timelogic hardware-accelerated boards. The best alignment against SILVA for each RNA sequence was extracted from the tera-blastn results. RNA sequences with alignments to rRNA in SILVA that had an e-value <1e −9 were discarded from further analyses, as they were assumed to be rRNA rather than mRNA. The mRNA nucleotide sequences reported in this paper have been deposited in the NCBI Short Read Archive: SRA058958. Read mapping of raw reads to contigs/ORFs RPKM values [23] , Reads Per Kilobase per Million mapped reads, for each DNA and mRNA sample were generated by the RNA-Seq Analysis pipeline in **CLC bio Genomics Workbench (version 4.7.2), and used to analyse contig and ORF frequency (DNA-RPKM) within the microbial community and also gene expression level (mRNA-RPKM, see below). All assembled metagenomic contigs (1,005,833), the longer contigs with a 500-bp length cutoff (224,995) and the related ORFs (445,806) were used as the references when mapping the raw reads against the metagenomic assemblies. The read mapping analysis in CLC bio Genomics Workbench was run with default settings, except for the use of 0.8 as the minimum length and the minimum similarity fractions ( Supplementary Table S2 ). The microbial composition within the community was analysed using the DNA frequency (DNA-RPKM) for each ORF. The entire collection of metagenomic ORFs yielded a DNA-RPKM value of 1,383,072, which was used in combination with the sum of RPKM values for each taxonomic group to describe relative taxonomic abundance within the microbial community. Bin-genome grouping for four abundant strains Bin-genomes, or draft genomes, were extracted by grouping the contigs of the estimated dominant strains within the anodic microbial community using four criteria: (i) predicted taxonomy of the contig, (ii) contig frequency as determined by DNA-RPKM, (iii) GC content and (iv) contig length. The specific values used for the bin-genome clustering are summarized in Supplementary Table S3 . To assess the genome ‘completeness’ of uncultured bacterial bin-genomes acquired from our metagenomic data sets, we used 107 marker genes for domain Bacteria ( Supplementary Table S4 ) ( [43] ) and 137 marker genes for domain Archaea ( Supplementary Table S5 ) ( [44] ) that were found to hit only one gene in >95% of nearly all bacterial/archaeal genomes as determined by KO functional annotation. The percentage of marker genes found in our bin-genomes was calculated and compared with that of completed genomes of closest relative strain(s). To assess the phylogenetic position of the bin-genomes, three peptide sequences ( gyrB , dsrA and mcrA ) were used to create phylogenetic trees by the neighbour-joining algorithms in the CLC Genomics Workbench version 5.0 (CLCbio). The detailed method is described in the Supplementary Methods . Functional gene families related to anaerobic respiration Approximately 40 gene families determined by KO were selected as targets to further analyse the different functions in the microbial community. These included ribosomal proteins, ftsZ gene, TCA cycle, NADH dehydrogenases, ATPases, multi-haem c- type cytochromes, dissimilatory sulphate reduction, methanogenesis and nitrate reduction ( Supplementary Table S7 ). The relative gene expression level for each gene family under each condition was determined by dividing the mRNA-RPKM by the DNA-RPKM (mRNA/DNA ratio). The specific gene expression dynamics that occurred as a function of condition change was determined by dividing the mRNA-RPKM of one condition by the mRNA-RPKM of the other condition (mRNA/mRNA ratio). The values were plotted in heatmap format using MATLAB (The MathWorks, Inc.). 16S rRNA clone analysis Total DNA for the three operational conditions was also used for 16S rRNA based clone analysis for both bacterial and archaeal communities. The detailed methods are described in Supplementary Methods . The nucleotide sequences reported in this paper have been deposited in the GSDB/DDBJ/EMBL/NCBI nucleotide sequence databases under accession numbers JX491497–JX491632. Quantitative PCR All PCR primers used for real-time PCR were designed by Primer 3 and synthesized at Integrated DNA Technologies. Target genes and respective primer sets are shown in Supplementary Table S8 . The detailed method for qPCR is described in Supplementary Methods . Accession codes: The assembled contigs from this metagenomic study have been deposited at DDBJ/EMBL/GenBank under the accession AMWB00000000. The version described in this paper is the first version, AMWB01000000, SRA058958 and JX491497-JX491632. How to cite this article: Ishii, S. et al. A novel metatranscriptomic approach to identify gene expression dynamics during extracellular electron transfer. Nat. Commun. 4:1601 doi: 10.1038/ncomms2615 (2013).